Endotrophin triggers adipose tissue fibrosis and metabolic dysfunction We recently identified endotrophin as an adipokine with potent tumour-promoting effects. However, the direct effects of local accumulation of endotrophin in adipose tissue have not yet been studied. Here we use a doxycycline-inducible adipocyte-specific endotrophin overexpression model to demonstrate that endotrophin plays a pivotal role in shaping a metabolically unfavourable microenvironment in adipose tissue during consumption of a high-fat diet (HFD). Endotrophin serves as a powerful co-stimulator of pathologically relevant pathways within the ‘unhealthy’ adipose tissue milieu, triggering fibrosis and inflammation and ultimately leading to enhanced insulin resistance. We further demonstrate that blocking endotrophin with a neutralizing antibody ameliorates metabolically adverse effects and effectively reverses metabolic dysfunction induced during HFD exposure. Collectively, our findings demonstrate that endotrophin exerts a major influence in adipose tissue, eventually resulting in systemic elevation of pro-inflammatory cytokines and insulin resistance, and the results establish endotrophin as a potential target in the context of metabolism and cancer. Excess caloric exposure along with insufficient energy expenditure is the main cause of the ongoing widespread obesity epidemic. The key tissue initially affected by over-nutrition is adipose tissue [1] , [2] . Indeed, whole-body metabolic homoeostasis depends critically on how well adipose tissue remodels in response to an excess of incoming calories [3] . Adipocytes and their progenitor cells (pre-adipocytes) are embedded in a loosely structured three-dimensional (3D) network of extracellular matrix (ECM) [4] . As a result, adipose tissue function is tightly regulated by its surrounding ECM proteins and their modifiers, for example, matrix metalloproteinases (MMPs). Fibrosis is a common pathological consequence of ECM dysregulation in many inflammatory diseases, defined by excess deposition of ECM proteins, especially proteins of the collagen family [5] . The pathological impact of the modulation of ECM rigidity and ensuing fibrosis on obesity and metabolism has been studied in depth in recent years [4] , [6] , [7] , [8] , [9] , [10] , [11] . Many studies have unveiled close links between the dynamics of ECM remodelling, the development of fibrosis and the pathogenesis of chronic inflammation in adipose tissue [8] , [12] . Adipose tissue-derived inflammation can exert a potent negative impact on systemic glucose tolerance, highlighted by recent data that demonstrated that selectively silencing inflammatory genes in epididymal adipose tissue macrophages leads to metabolic improvements [13] . Particularly the MMPs play an important role in this process leading up to inflammation. As an example, a dramatic phenotype is seen in the absence of MTP1-MMP (MMP14). In this setting, the rigidity of ECM in the developing subcutaneous fat pads increases due to abnormal accumulation of collagens. This developmental fibrotic response in turn leads to limited adipose expansion, and prompts complete lipodystrophy [4] . In contrast, when the COL6 −/− mouse was crossed onto an ob/ob background, the weakened ECM in COL6 −/− ob/ob adipose tissue enables the adipocytes to expand unhindered, without the associated necrosis and inflammation conventionally seen under these conditions. Consequently, the mice remain more insulin sensitive compared with their littermate ob/ob controls due to this ‘healthy’ expansion [7] . Clinically, in obese human adipose tissue, large areas of fibrosis can be found; these areas contain elevated levels of COL6, along with infiltration of many classically activated (M1) macrophages [14] , [15] . COL6 is an abundant constituent of white adipose tissue (WAT) [6] , [7] , [15] , [16] . In fact, it is the most highly expressed collagen in differentiated adipocytes and undergoes significant structural remodelling during adipogenesis [7] . Of note, several studies have demonstrated that COL6 levels positively correlate with hyperglycaemia and insulin resistance [17] , [18] , suggesting an important metabolic role in adipose tissue. COL6 is composed of three distinct α chains, α1, α2 and α3. These chains fold together to form COL6 trimeric building block. The trimers further assemble into trimer-dimers and trimer-tetramers, and are subsequently secreted into the ECM where they eventually organize into mature microfibrils [19] , [20] . Specifically, the α3 chain, by far the longest of the three chains, contains an unusually long N terminus and a globular C5 domain at the C-terminus. The C-terminal portion of the α3 subunit is cleaved off during the post-translational processing of COL6 fibrils. However, the time-point and location of the cleavage process, the specific MMP(s) involved and the exact cleavage event within the α3 chain remain to be defined in detail [21] . We recently followed up on the studies of the C-terminal cleavage product involving this C5 domain of COL6α3 (that we referred to as endotrophin). With a specific antibody we generated, we detected abundant secretion of endotrophin from fully differentiated 3T3-L1 adipocytes but not in the preadipocytes [22] . We further observed that endotrophin is upregulated in ob/ob fat pads compared with those in lean littermates [22] . More importantly, we demonstrated that endotrophin within the tumour microenvironment serves as a major mediator of COL6-stimulated mammary tumour growth and subsequent chemoresistance [22] , [23] . Specifically, endotrophin stimulates fibrosis, activates endothelial cell migration and promotes macrophage infiltration into growing solid tumours. All these steps ultimately lead to elevated mammary tumour expansion and more pronounced metastatic growth [22] . While the crucial function of endotrophin in tumour development has been characterized, as an adipocyte-derived and an obesity-associated factor, its direct action in adipose tissue dysfunction in the absence of an infiltrating tumour remains to be elucidated. We hypothesized that endotrophin induced by obesity may not only be associated with adipose tissue fibrosis, macrophage chemotaxis, inflammation and an unfavourable metabolic profile, but rather, endotrophin could be a driving factor for this process. To test this hypothesis in the present study, we used a doxycycline (Dox)-inducible adipose tissue-specific endotrophin overexpression model. Gene expression profiling indicates that endotrophin overexpression upregulates pro-fibrotic and pro-inflammatory genes in fat pads of the transgenic mice. Specifically, under a high-fat diet (HFD) challenge, endotrophin serves as a powerful co-stimulator of existing pathological processes within the ‘unhealthy’ adipose tissue milieu to trigger further enhancement of fibrosis and inflammation, leading to increased insulin resistance. Consistent with its role as a necessary and sufficient factor worsening the pathological response to a dietary intervention in a diet-induced obese (DIO) model, we further demonstrate that a neutralizing antibody against endotrophin ameliorates the metabolically adverse effects induced by HFD. Collectively, our findings highlight endotrophin as an important adipokine that exerts a major influence locally in adipose tissue, mediating a systemic elevation of pro-inflammatory cytokines and insulin resistance in many other tissues. Generation of endotrophin-overexpressing transgenic mice COL6 is composed of three subunits: COL6α1, COL6α2 and COL6α3. Endotrophin is the C5 domain of COL6α3 ( Supplementary Fig. 1A , highlighted in red). Compared with the stromal–vascular fractions, the expression levels of all three subunits were significantly higher in adipocytes ( Fig. 1a ). This prompted us to choose an adipocyte-specific overexpression model for endotrophin in the context of metabolic analysis. To assess the function of endotrophin locally in adipose tissue, we established a double transgenic mouse strain employing a tetracycline-inducible system. Supplementary Fig. 1B shows a schematic representation of this mouse model. We have previously described our adipocyte-specific tetracycline response element-driven (TRE) system [24] . In this model, the TRE promoter is regulated by the reverse tetracycline-dependent transcriptional activator (rtTA), whose expression is under the control of the adipose tissue-specific adiponectin promoter [25] . In this case, we used the system to drive expression of endotrophin fused to a prolactin signal sequence at its N terminus to ensure that the overexpressed endotrophin can be secreted [22] . This allows us to probe for a physiologically relevant local elevation of endotrophin without a concomitant overexpression of the full-length version of COL6α3 or its combination with COL6α1, COL6α2. In these initial studies, we performed a very acute induction of endotrophin for just 5 days on normal chow containing 600 mg kg −1 Dox. The endotrophin mRNA levels were induced in different adipose tissues, especially in mesenteric WAT, subcutaneous WAT (SWAT) and brown adipose tissue (BAT) ( Fig. 1b ), whereas no induction was observed in other tissues or in the absence of Dox treatment ( Fig. 1b ). Immunohistochemical staining with anti-mouse endotrophin antibodies demonstrates the overexpression at the protein level in epididymal WAT (EWAT) of endotrophin transgenic mice ( Fig. 1c ). Even under these short-term exposure times, the genes that potentially are affected by endotrophin overexpression, such as COL3α1 and COL6α1 were indeed both significantly upregulated in SWAT of the endotrophin transgenic mice. Other related genes, such as COL1α1, LOX and F4/80, also showed strong trends towards a transcriptional increase ( Fig. 1d ). 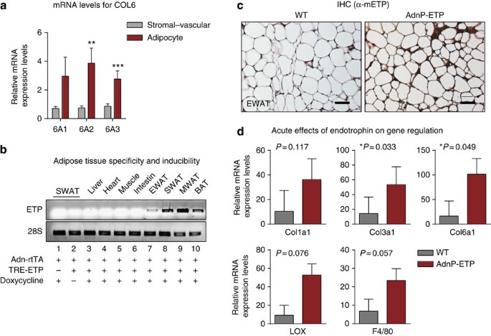Figure 1: Endotrophin expression in AT induces fibrosis and inflammation-related genes in WAT. (a) Q–PCR analysis for stromal–vascular versus adipocyte distribution of Col6 mRNAs. Data represents mean±s.d. (n=5). **P<0.01 and ***P<0.001 versus stromal-vesicular by two-way analysis of variance. (b) PCR analysis of endotrophin overexpression in different fat pads (EWAT (epididymal), SWAT (subcutaneous), MWAT (mesenteric) and BAT (brown adipose tissue) and other organs in the adiponectin promoter-driven TRE-ETP (AdnP-ETP) transgenic mice and their littermate controls 5 days after Dox induction on a chow diet (n=5 per group). (c) Immunohistochemical staining with an anti-mouse endotrophin antibody of EWAT from the transgenic mice and their littermate controls. Scale bar, 100 μm. (d) Q–PCR analysis of pro-fibrotic and pro-inflammatory genes affected by endotrophin overexpression in SWAT of the transgenic mice and their littermate controls 5 days after Dox induction (n=5 per group, Student’st-test for all theP-values). Figure 1: Endotrophin expression in AT induces fibrosis and inflammation-related genes in WAT. ( a ) Q–PCR analysis for stromal–vascular versus adipocyte distribution of Col6 mRNAs. Data represents mean±s.d. ( n =5). ** P <0.01 and *** P <0.001 versus stromal-vesicular by two-way analysis of variance. ( b ) PCR analysis of endotrophin overexpression in different fat pads (EWAT (epididymal), SWAT (subcutaneous), MWAT (mesenteric) and BAT (brown adipose tissue) and other organs in the adiponectin promoter-driven TRE-ETP (AdnP-ETP) transgenic mice and their littermate controls 5 days after Dox induction on a chow diet ( n =5 per group). ( c ) Immunohistochemical staining with an anti-mouse endotrophin antibody of EWAT from the transgenic mice and their littermate controls. Scale bar, 100 μm. ( d ) Q–PCR analysis of pro-fibrotic and pro-inflammatory genes affected by endotrophin overexpression in SWAT of the transgenic mice and their littermate controls 5 days after Dox induction ( n =5 per group, Student’s t- test for all the P -values). Full size image Endotrophin in adipose tissue causes metabolic dysregulation To investigate the metabolic consequences of a more chronic endotrophin overexpression in adipose tissue, the transgenic mice and wild-type littermate controls were challenged with HFD plus 600 mg kg −1 Dox for 8 weeks. During the 8-week HFD exposure, endotrophin-expressing mice gained slightly more weight ( Fig. 2a ). Despite the only moderately elevated weights, the transgenic mice displayed significantly elevated serum triglycerides ( Fig. 2b ) and non-esterified free fatty acids ( Fig. 2c ). This was paralleled by a significantly enhanced accumulation of hepatic triglyceride ( Fig. 2d ) and with an increase in hepatic cholesterol levels as well ( Fig. 2e ). This is not surprising in light of the fact that once a significant local level of dysfunction is established in adipose tissue, adipocytes can no longer effectively fulfil their role as lipid-sinks, and lipids start to build up ectopically in other tissues [26] . In line with the biochemical data, liver histology revealed an increase in lipid droplet number and size ( Fig. 2f ), demonstrating a severe liver steatosis in the transgenic animals. Overexpression of endotrophin thus, to a large extent, results in abnormal lipid metabolism and hence causes ectopic steatosis. We conclude that overexpression of endotrophin specifically in adipose tissue impairs proper function of adipocytes and hence brings about systemic metabolic dysfunction. This is apparent when oral glucose tolerance tests (OGTTs) and insulin sensitivity tests (ITTs) are performed ( Fig. 2g,h ). Endotrophin overexpressing mice display a larger area under the curve for the OGTT, and show a less significant decrease in plasma glucose levels upon injection of insulin during an ITT. Furthermore, adipokines, such as adiponectin and leptin, are mediators linking adipose tissue metabolism to inflammation and immunity [27] . Q–PCR shows that mRNA levels of adiponectin had a trend towards a decrease, whereas leptin had a trend to increase in SWAT of endotrophin transgenic mice ( Supplementary Fig. 2A ). As a result, circulating adiponectin levels are significantly decreased, whereas leptin levels in serum are significantly increased in endotrophin transgenic mice ( Supplementary Fig. 2B,C ). 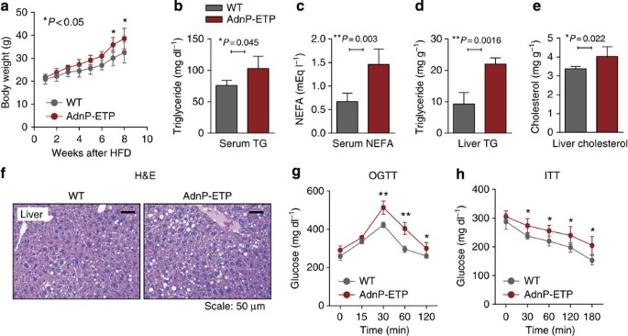Figure 2: Overexpression of endotrophin locally in adipose tissue promotes metabolic dysfunction under a HFD challenge. (a) Body weight gain in endotrophin transgenic mice and their littermate controls during HFD plus 600 mg kg−1Dox treatment for 8 weeks (n=5 per group, Student’st-test for all theP-values). (b) Serum TG and (c) NEFA levels in endotrophin transgenic mice and their littermate controls after HFD plus Dox treatment for 8 weeks (n=5 per group, Student’st-test for all theP-values). (d) Liver TG and (e) cholesterol levels in endotrophin transgenic mice and their littermate controls after HFD plus Dox treatment for 8 weeks (n=4 for control;n=5 for endotrophin Tg, Student’st-test for all theP-values). (f) H&E staining of liver sections from endotrophin transgenic mice and their littermate controls 8 weeks after HFD plus Dox treatment. Scale bars, 50 μm. (g) Blood glucose levels during an OGTT and an ITT in endotrophin transgenic mice and their littermate controls after HFD plus Dox treatment for 5 weeks (n=5 for each group, Student’st-test for all theP-values). (h) Blood glucose levels during an ITT in endotrophin transgenic mice and their littermate controls after HFD plus Dox treatment for 5 weeks (n=5 for each group, Student’st-test for all theP-values). Figure 2: Overexpression of endotrophin locally in adipose tissue promotes metabolic dysfunction under a HFD challenge. ( a ) Body weight gain in endotrophin transgenic mice and their littermate controls during HFD plus 600 mg kg −1 Dox treatment for 8 weeks ( n =5 per group, Student’s t- test for all the P -values). ( b ) Serum TG and ( c ) NEFA levels in endotrophin transgenic mice and their littermate controls after HFD plus Dox treatment for 8 weeks ( n =5 per group, Student’s t -test for all the P -values). ( d ) Liver TG and ( e ) cholesterol levels in endotrophin transgenic mice and their littermate controls after HFD plus Dox treatment for 8 weeks ( n =4 for control; n =5 for endotrophin Tg, Student’s t -test for all the P -values). ( f ) H&E staining of liver sections from endotrophin transgenic mice and their littermate controls 8 weeks after HFD plus Dox treatment. Scale bars, 50 μm. ( g ) Blood glucose levels during an OGTT and an ITT in endotrophin transgenic mice and their littermate controls after HFD plus Dox treatment for 5 weeks ( n =5 for each group, Student’s t- test for all the P -values). ( h ) Blood glucose levels during an ITT in endotrophin transgenic mice and their littermate controls after HFD plus Dox treatment for 5 weeks ( n =5 for each group, Student’s t -test for all the P -values). Full size image Endotrophin triggers local inflammation in adipose tissue To further explore the adverse effects of endotrophin overexpression in adipose tissue, we sought to determine whether endotrophin can trigger fibrosis and pathological ECM expansion during HFD exposure, in similar ways we have previously observed in the context of endotrophin-expressing mammary tumours. Q–PCR analysis of adipose tissue demonstrated that several ECM markers were upregulated after 8 weeks of Dox induction ( Fig. 3a ). COL3α1 and COL6α1, two major components of ECM in adipose tissue, were upregulated in SWAT of endotrophin transgenic mice as was the matrix metalloprotease MMP12. Interestingly, TGF-β1 and its receptor 2 (TGF-β R2) levels were also significantly increased in adipose tissue of the transgenic mice, consistent with our previous observations in tumour tissue that suggested that the activation of the TGF-β pathway is an integral part of endotrophin’s fibrotic effects [22] . 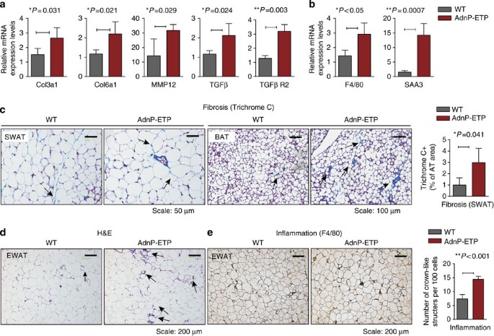Figure 3: Overexpression of endotrophin locally in adipose tissue stimulates fibrosis and exacerbates inflammation induced by HFD. (a) Q–PCR analysis for collagen 3α1 and 6α1, TGFβ and its receptor (TGFβ R2) and MMP12 in SWAT of endotrophin transgenic mice and their littermate controls (n=4 for each group, Student’st-test for all theP-values) after 8 weeks of exposure to HFD plus Dox. (b) Q–PCR analysis for adipose tissue inflammation-related genes F4/80 and SAA3 in SWAT of endotrophin transgenic mice and their littermate controls (n=4 for each group, Student’st-testfor both theP-values). (c) A Masson’s trichrome stain of SWAT (left panels) and BAT (right panels) from endotrophin transgenic mice and their littermate controls. Scale bars, 50 μm for SWAT and 100 μm for BAT. The right panel shows the quantitative measurements of the stain in SWAT by ImageJ software (Student’st-test,P=0.041). (d) H&E staining of EWAT from endotrophin transgenic mice and their littermate controls. The arrows point to the CLS formed by macrophage aggregation in HFD-fed mice. Scale bars, 200 μm. (e) Immunohistochemical staining of F4/80 in EWAT from endotrophin transgenic mice and their littermate controls (left panels). Note the CLS formed by macrophage aggregation in HFD-fed mice. The right panel shows quantitative measurements of the numbers of CLS (n=5 per group, Student’st-test,P<0.001). Scale bar, 200 μm. Figure 3: Overexpression of endotrophin locally in adipose tissue stimulates fibrosis and exacerbates inflammation induced by HFD. ( a ) Q–PCR analysis for collagen 3α1 and 6α1, TGFβ and its receptor (TGFβ R2) and MMP12 in SWAT of endotrophin transgenic mice and their littermate controls ( n =4 for each group, Student’s t- test for all the P -values) after 8 weeks of exposure to HFD plus Dox. ( b ) Q–PCR analysis for adipose tissue inflammation-related genes F4/80 and SAA3 in SWAT of endotrophin transgenic mice and their littermate controls ( n =4 for each group, Student’s t-test for both the P -values). ( c ) A Masson’s trichrome stain of SWAT (left panels) and BAT (right panels) from endotrophin transgenic mice and their littermate controls. Scale bars, 50 μm for SWAT and 100 μm for BAT. The right panel shows the quantitative measurements of the stain in SWAT by ImageJ software (Student’s t- test, P =0.041). ( d ) H&E staining of EWAT from endotrophin transgenic mice and their littermate controls. The arrows point to the CLS formed by macrophage aggregation in HFD-fed mice. Scale bars, 200 μm. ( e ) Immunohistochemical staining of F4/80 in EWAT from endotrophin transgenic mice and their littermate controls (left panels). Note the CLS formed by macrophage aggregation in HFD-fed mice. The right panel shows quantitative measurements of the numbers of CLS ( n =5 per group, Student’s t -test, P <0.001). Scale bar, 200 μm. Full size image As inflammation has been reported to be a late-stage phenomenon of fibrosis in adipose tissue [1] , we further determined whether endotrophin expression exacerbates inflammation induced by HFD. Indeed, we found that mRNA levels of both the macrophage marker F4/80 and the acute-phase inflammatory marker serum amyloid A3 (SAA3) were significantly increased in endotrophin transgenic mice after 8 weeks of Dox induction ( Fig. 3b ). Consistent with the ECM gene expression analysis, histological examination of both SWAT and BAT with a Masson’s trichrome stain showed that the extracellular matrix accumulation was elevated in the transgenic mice as judged by the dense blue stain in the transgenic adipose tissues ( Fig. 3c ). In line with the upregulation of inflammatory markers, H&E staining indicates that there is a higher frequency of immune cell infiltration into the transgenic fat pads judged by the ‘crown-like’ structures surrounding adipocytes in EWAT of endotrophin transgenic mice ( Fig. 3d ). Immunohistochemical analysis with an anti-macrophage antibody (anti-F4/80) confirms an increased level of macrophages in the ‘crown-like’ structures in the endotrophin transgenic mice, presumably surrounding dead adipocytes, apparent when examined visually and even more apparent upon quantitation ( Fig. 3e ). This suggests that chronic local overexpression of endotrophin in adipose tissue stimulates fibrosis and inflammation. Unique effects of endotrophin on the intradermal fat layer Although there were significant changes in fat pads in some of the parameters that we reported above, overall there were minimal effects on individual fat pad weights and average size of the adipocytes. One major exception to this is the intradermal fat layer, which usually consists of a layer of adipocytes less than a dozen cells thick. Endotrophin-overexpressing mice display a dramatic increase in the depth of this intradermal fat layer ( Supplementary Fig. 3 ). However, this is at the expense of the dermal thickness, which is reduced in the transgenic animals. Although the underlying mechanism or teleological reason for the hyperproliferation of this intradermal fat layer remain unknown, the increase in this gain-of-function setting for endotrophin is consistent with the complete disappearance of adipocytes in this layer in the context of the functional collagen 6 knockout that we previously reported [7] . Endotrophin in adipose tissue leads to lower energy expenditure To determine whether dysfunction of BAT caused by fibrosis affects systemic metabolism, we monitored the energy expenditure in the endotrophin transgenic mice and their littermate controls in metabolic chambers. The oxygen consumption rate (VO 2 ) ( Supplementary Fig. 4A ) and VCO 2 ( Supplementary Fig. 4B ) were both significantly reduced in endotrophin transgenic mice, reflecting a decrease in energy expenditure. In contrast, the overall respiratory exchange rate (RER) displayed no changes ( Supplementary Fig. 4C ), suggesting no substrate preference in the transgenic mice compared with wild-type littermates. Food intake was comparable within the accuracy of our measurements ( Supplementary Fig. 4E ). Heat generation within the cages was significantly lower in the transgenic mice ( Supplementary Fig. 4D ). These observations at least partially explain the increased body weight gain in the transgenic mice on HFD on the basis of reduced energy expenditure. Note that these measurements were performed at 6 weeks of HFD exposure before the point when the body weights significantly differed. Suppression of endotrophin improves insulin sensitivity We have previously generated a rat anti-mouse endotrophin antibody that neutralizes endotrophin activity. We have shown that this antibody effectively reduced the growth of a mammary tumour mass infiltrating the mammary fat pad, reduced the number of metastatic lesions [22] and enhanced chemosensitivity of tumour cells [23] . The therapeutic potential of these endotrophin-neutralizing monoclonal antibodies on metabolic and fibrotic parameters have not yet been established. DIO mice were treated twice a week with intraperitoneal (i.p.) injections of either an isotype-adjusted IgG control or the monoclonal anti-mouse endotrophin antibody, clone 10B6. Treatment with antibodies was started 2 weeks after initiation of the HFD challenge in this case, and was maintained for another 4 weeks while the animals were kept on the HFD. So we allowed the dietary challenge to establish a metabolic insult, though only for 2 weeks, and maintained this challenge during the antibody treatment. Body weights were not different among the treatment and control groups ( Fig. 4a ). Furthermore, DIO mice exposed to 10B6 displayed improved levels of serum triglycerides ( Fig. 4b ) (113±21 mg dl −1 in isotype IgG- and 44±5 mg dl −1 in 10B6-treated mice, unpaired Student’s t -test, P =0.0283) and free fatty acids ( Fig. 4c ) (1.18±0.27 mEq l −1 in IgG- and 0.41±0.03 mEq l −1 in 10B6-treated mice, unpaired Student’s t -test, P =0.04), whereas the serum cholesterol levels were not affected by endotrophin neutralization ( Fig. 4d ) (unpaired Student’s t -test, P =NS). Similarly, the levels of hepatic triglycerides were also improved ( Fig. 4e ) (22.5±3.4 mg g −1 in isotype IgG versus 13.4±0.1 mg g −1 in 10B6-treated mice; unpaired Student’s t -test, P =0.035), whereas the cholesterol levels were comparable between the two groups ( Fig. 4f , unpaired Student’s t -test, P =NS). Consistent with the biochemical data, histological analysis of H&E-stained liver sections indicated that hepatic lipid accumulation in DIO mice was significantly reduced in 10B6 treatment compared with isotype IgG controls ( Fig. 4g ). 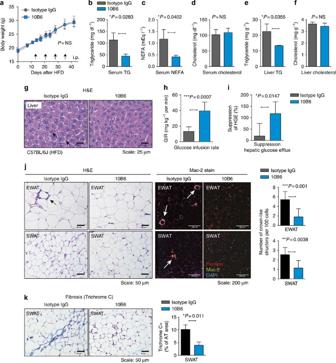Figure 4: Endotrophin neutralization improves metabolic dysfunction. (a) Two cohorts of mice (n=8) were exposed to HFD for 45 days after weaning. At the indicated time points (arrowheads), mice were treated with anti-endotrophin monoclonal antibodies (100 μg per mouse) or equivalent amounts of non-immune antibody. Body weights were monitored. (b) Plasma triglycerides; (c) plasma free fatty acids (NEFAs); (d) plasma cholesterol; (e) hepatic triglycerides; (f) hepatic cholesterol. Significant differences as indicated by unpaired Student’st-test. (g) Hepatic histology (H&E stain) reveals clear differences in hepatic lipid accumulation. Scale bar, 25 μm. (h) Glucose infusion rate and (i) Suppression of hepatic glucose efflux was measured during a hyperinsulinemic–euglycemic clamp. Significant differences as indicated by unpaired Student’st-test. (j) Left: H&E staining of EWAT and SWAT in either isotype IgG- or 10B6-treated HFD-induced obese mice. Scale bar, 50 μm. Quantification for CLS in EWAT and SWAT represents mean±s.d. (three different fields fromn=5 per group). Significant differences as indicated by unpaired Student’st-test. Right: Mac-2 immunostaining of EWAT and SWAT, showing decreased inflammation in 10B6-given mice compared with IgG control. Adipocyte membrane and nucleus were visualized by co-staining with anti-perilipin and DAPI. Scale bar, 200 μm. (k) Masson’s trichrome C staining of SWTA shows decreased fibrosis in SWAT in 10B6-given mice compared with IgG control. Quantification for the area of TC positive stains in SWAT represents mean±s.d. (three different fields fromn=5 per group). Significant differences as indicated by unpaired Student’st-test. Scale bar, 50 μm. Figure 4: Endotrophin neutralization improves metabolic dysfunction. ( a ) Two cohorts of mice ( n =8) were exposed to HFD for 45 days after weaning. At the indicated time points (arrowheads), mice were treated with anti-endotrophin monoclonal antibodies (100 μg per mouse) or equivalent amounts of non-immune antibody. Body weights were monitored. ( b ) Plasma triglycerides; ( c ) plasma free fatty acids (NEFAs); ( d ) plasma cholesterol; ( e ) hepatic triglycerides; ( f ) hepatic cholesterol. Significant differences as indicated by unpaired Student’s t -test. ( g ) Hepatic histology (H&E stain) reveals clear differences in hepatic lipid accumulation. Scale bar, 25 μm. ( h ) Glucose infusion rate and ( i ) Suppression of hepatic glucose efflux was measured during a hyperinsulinemic–euglycemic clamp. Significant differences as indicated by unpaired Student’s t -test. ( j ) Left: H&E staining of EWAT and SWAT in either isotype IgG- or 10B6-treated HFD-induced obese mice. Scale bar, 50 μm. Quantification for CLS in EWAT and SWAT represents mean±s.d. (three different fields from n =5 per group). Significant differences as indicated by unpaired Student’s t -test. Right: Mac-2 immunostaining of EWAT and SWAT, showing decreased inflammation in 10B6-given mice compared with IgG control. Adipocyte membrane and nucleus were visualized by co-staining with anti-perilipin and DAPI. Scale bar, 200 μm. ( k ) Masson’s trichrome C staining of SWTA shows decreased fibrosis in SWAT in 10B6-given mice compared with IgG control. Quantification for the area of TC positive stains in SWAT represents mean±s.d. (three different fields from n =5 per group). Significant differences as indicated by unpaired Student’s t -test. Scale bar, 50 μm. Full size image To examine the effects of endotrophin neutralization on insulin sensitivity, we performed hyperinsulinemic–euglycemic clamps on DIO mice given either isotype IgG or 10B6. Strikingly, 10B6-treated DIO mice improved whole-body insulin sensitivity, as determined by the glucose infusion rate required to maintain euglycemia ( Fig. 4h ) and by the amount of suppression of hepatic glucose efflux ( Fig. 4i and Table 1 ). Collectively, these data from a DIO setting suggest that endotrophin neutralization by 10B6 monoclonal antibody improves metabolic profiles, resulting in enhanced lipid and carbohydrate handling, as judged by plasma parameters such as the levels of circulating triglyceride and free fatty acids, as well as by measuring hepatic triglycerides and hepatic glucose output leading to an increase in whole-body insulin sensitivity. This highlights the therapeutic potential of this approach. Table 1 Parameters before and during hyperinsulinemic–euglycemic clamp studies. Full size table Endotrophin neutralization attenuates adipose tissue inflammation Endotrophin augments tissue fibrosis, inflammation and angiogenesis in the context of a tumour infiltrating into adipose tissue [22] . All of these phenomena are also well-established contributors to insulin resistance and generalized adipose tissue dysfunction. As endotrophin neutralization improves whole-body insulin sensitivity in DIO mice, we also examined various adipose tissue depots in DIO mice with respect to tissue fibrosis, inflammation and angiogenesis after neutralizing antibody treatment in the same cohort of mice. Histological analysis indicated that the most striking differences were observed at the level of chronic inflammation in both EWAT and SWAT, as well as tissue fibrosis in both SWAT and BAT. More specifically, DIO-induced chronic inflammation in EWAT and SWAT was significantly decreased by 10B6 treatment, as judged by counting numbers of ‘crown-like structures’ (CLS) in adipose tissues ( Fig. 4j ), a reflection of dysfunctional or dead adipocytes. These observations were further confirmed with immunostaining for the macrophage-specific Mac-2 marker, indicating that macrophage accumulation in adipose tissues upon DIO exposure is significantly suppressed by 10B6 treatment, particularly in EWAT and SWAT. Tissue fibrosis was significantly protected by 10B6 treatment particularly in SWAT where fibrosis is prone to be placed upon DIO, as quantified by a positive area of Masson’s trichrome C stains ( Fig. 4k ). In contrast, 10B6 treatment seemed to have a limited effect on angiogenesis in adipose tissues as determined by a lectin perfusion ( Supplementary Fig. 5 ). Endotrophin neutralization after HFD The initial cohort analysed in Fig. 4 was challenged for 2 weeks before antibody treatment initiation. We wanted to test whether the neutralizing antibody would retain a therapeutic potential even after prolonged HFD exposure. We therefore repeated the experiment in Fig. 4 on two additional cohorts that were challenged for up to 10 weeks with a HFD, and antibody treatment was then initiated for an additional 3.5 weeks on the HFD. With both independent cohorts, we obtained comparable results, and we are showing the results of one of these cohorts in Fig. 5 . Even after prolonged HFD pretreatment ( Fig. 5a ), endotrophin neutralization had a significant effect on the number of CLSs that were histologically apparent by H&E in EWAT and SWAT, with even more significant differences than were apparent after the shorter HFD exposure ( Fig. 5b ). These findings were further substantiated with a macrophage-specific Mac-2 stain ( Fig. 5c ), showing a substantial reduction in overall Mac-2 signal observed in both EWAT and SWAT. Lipid droplet accumulation in the liver was reduced under these conditions, suggesting a dramatic reduction of hepatic steatosis ( Fig. 5d ). No effects on body weight or baseline glucose levels were observed, similar to the other experiments reported in Fig. 4 . However, these histological improvements result in a significant improvement of an OGTT in agreement with the detailed clamp studies in Fig. 4 and Table 1 , suggesting enhanced hepatic insulin sensitivity. Combined, these results suggest that the neutralization of endotrophin effectively improves adipose tissue health and the systemic metabolic profile even after prolonged HFD exposure. 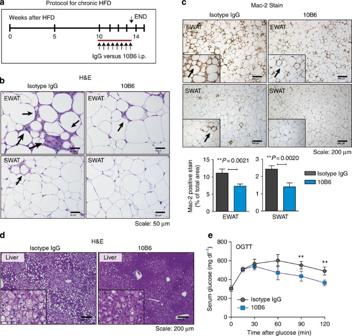Figure 5: Histological analysis of AT following endotrophin neutralization after chronic HFD exposure. (a) The schematic representation of the protocol for chronic HFD experiments. (b) H&E staining of EWAT and SWAT in either isotype IgG- or 10B6-treated HFD mice (8 weeks of HFD pre-treatment before initiation of antibody treatment). Scale bar, 50 μm. Quantification for CLS in EWAT and SWAT represents mean±s.d. (three different fields fromn=5 per group). Significant differences as indicated by unpaired Student’st-test. (c) Mac-2 immunostaining of EWAT and SWAT, showing decreased inflammation in 10B6-given mice compared with IgG control. Adipocyte membrane and nucleus were visualized by co-staining with anti-perilipin and DAPI. Scale bar, 200 μm. (d) Hepatic histology (H&E stain) reveals differences in hepatic lipid accumulation. Scale bar, 200 μm. (e) C57/Bl6J mice were challenged with HFD for 8 weeks and subsequently treated with either 10B6 (100 μg per mouse, twice weekly by IP) or IgG control for another 3 weeks. OGTT was performed. Serum glucose levels during OGTT. Data represents mean±s.d. (n=6 per group). **P<0.01 versus IgG by multiplet-tests. Figure 5: Histological analysis of AT following endotrophin neutralization after chronic HFD exposure. ( a ) The schematic representation of the protocol for chronic HFD experiments. ( b ) H&E staining of EWAT and SWAT in either isotype IgG- or 10B6-treated HFD mice (8 weeks of HFD pre-treatment before initiation of antibody treatment). Scale bar, 50 μm. Quantification for CLS in EWAT and SWAT represents mean±s.d. (three different fields from n =5 per group). Significant differences as indicated by unpaired Student’s t -test. ( c ) Mac-2 immunostaining of EWAT and SWAT, showing decreased inflammation in 10B6-given mice compared with IgG control. Adipocyte membrane and nucleus were visualized by co-staining with anti-perilipin and DAPI. Scale bar, 200 μm. ( d ) Hepatic histology (H&E stain) reveals differences in hepatic lipid accumulation. Scale bar, 200 μm. ( e ) C57/Bl6J mice were challenged with HFD for 8 weeks and subsequently treated with either 10B6 (100 μg per mouse, twice weekly by IP) or IgG control for another 3 weeks. OGTT was performed. Serum glucose levels during OGTT. Data represents mean±s.d. ( n =6 per group). ** P <0.01 versus IgG by multiple t- tests. Full size image Endotrophin levels are higher in diabetic human patients Previously, we generated an anti-human endotrophin polyclonal antibody and used this antibody to investigate endotrophin levels in tumour cells. These studies revealed a strong upregulation of the protein in the tumour microenvironment, with a high affinity of endotrophin for tumour cells. Here, we wanted to test the expression in human adipocytes under normal and metabolically challenged conditions. Our initial experiments focused on immunofluorescent studies of mature human adipocytes. COL6 is abundantly expressed by human adipocytes as well as in the vascular endothelium of blood vessels. Staining against the cleaved endotrophin molecule reveals a distinct pattern at the level of the plasma membrane and secretory vesicles. The majority of endotrophin is located outside the adipocyte plasma membrane. Interestingly, and in line with previous observations, there is essentially no overlap between the mature COL6 fibrils and the C-terminal endotrophin fragment ( Supplementary Fig. 6A ). Moreover, immunofluorescent co-stains reveal that there is also essentially no co-localization between endotrophin and many other adipose proteins, such as adiponectin, leptin, BiP, caveolin-1 and GLUT4, further underlining the distinct ECM localization of endotrophin ( Supplementary Fig. 6B ). In contrast, under the conditions chosen, there is substantial overlap of GLUT4 with IRAP (insulin-responsive aminopeptidase), which has been included as a positive control to demonstrate co-localization of two established markers. The unique dotted staining pattern of endotrophin further supports its extracellular accumulation, which is distinct from its parental COL6 chains. We also wanted to test whether endotrophin upregulation in adipose tissue is strictly a function of obesity, or whether the relative metabolic fitness of the adipose tissue makes a difference, that is, would obese individuals with a low HOMA2-IR index have lower than expected levels of endotrophin, given their body mass index (BMI). For this purpose, endotrophin immunostaining was performed on human mesenteric adipose tissue from BMI-matched individuals with either normal insulin sensitivity (HOMA2-IR<1.7) or a HOMA2-IR>2.6. The endotrophin protein signal was integrated across 31 such specimens. The groups are comparable for BMI, age and glycaemia. There is no difference between the two groups in the number of diabetics ( Supplementary Table 2 ). The group of individuals with HOMA2-IR>2.6 displayed higher levels of endotrophin. Both groups included some individuals with frank diabetes, so the increase in endotrophin signal is more likely associated with the reduced insulin sensitivity, rather than fasting glucose levels which are comparable between the two groups ( Fig. 6a ). Furthermore, we complemented these stains with a generic analysis of overall fibrotic content of the tissues with a trichrome stain. This also demonstrated increased overall fibrosis in metabolically challenged obese adipose tissue as opposed to obese adipose tissue associated with normal metabolic function ( Fig. 6b ). 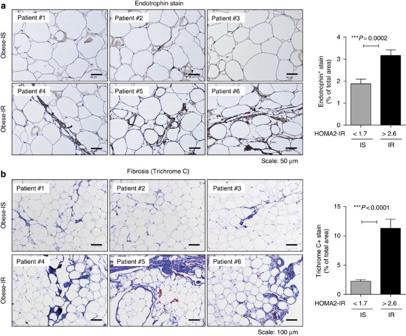Figure 6: Endotrophin is upregulated in fat tissue from obese human subjects with HOMA-IR>2.6. (a) Human subcutaneous adipocytes from healthy obese (normal HOMA-IR) and obese patients with HOMA-IR>2.6 were stained with a polyclonal antibody that specifically recognizes human endotrophin. Scale bar, 50 μm. The right panel indicates the quantitative measurement of anti-endotrophin positive stains by ImageJ software from NIH (Student’st-test for theP-value). (b) Human subcutaneous adipocytes from the same cohort as inawere stained with Masson’s trichrome C. Scale bar, 100 μm. The right panel indicates the quantitative measurement of the trichrome C positive signal by ImageJ software from NIH (Student’st-test for theP-value). Figure 6: Endotrophin is upregulated in fat tissue from obese human subjects with HOMA-IR>2.6. ( a ) Human subcutaneous adipocytes from healthy obese (normal HOMA-IR) and obese patients with HOMA-IR>2.6 were stained with a polyclonal antibody that specifically recognizes human endotrophin. Scale bar, 50 μm. The right panel indicates the quantitative measurement of anti-endotrophin positive stains by ImageJ software from NIH (Student’s t- test for the P -value). ( b ) Human subcutaneous adipocytes from the same cohort as in a were stained with Masson’s trichrome C. Scale bar, 100 μm. The right panel indicates the quantitative measurement of the trichrome C positive signal by ImageJ software from NIH (Student’s t -test for the P -value). Full size image Previous studies have demonstrated that excess caloric intake initiates rapid expansion of fat pads, which leads very quickly to a state of hypoxia in adipose tissue [1] , [28] , [29] , [30] , [31] . Hypoxia in metabolically challenged adipose tissue further leads to a fibrotic response by upregulating many ECM proteins, including collagens and collagen cross-linking enzymes, such as lysyl oxidase (LOX) [29] , [32] . Adipose tissue fibrosis is associated with a rigid ECM environment. This mechanical stress restrains further adipocyte expansion and leads to an increased frequency of adipocyte cell death and an enhanced inflammatory response [1] . Among the pro-fibrotic constituents, COL6 is an abundant local contributor to the ECM milieu of adipose tissue [7] . Specifically, a cleaved product from the C5 domain of COL6α3 chain (endotrophin) is upregulated in obese fat pads and in malignant tumours [6] , [22] . Recently, we demonstrated that overexpression of endotrophin in the tumour stroma stimulates fibrosis, angiogenesis and inflammation. These phenomena are thought to be triggered by endotrophin action through increased fibrogenesis, a stimulation of epithelial–mesenchymal transition and enhanced chemo-attraction of macrophages and endothelial precursor cells [22] . In the current study, we are starting to characterize the local effects of endotrophin on fat tissue by using a transgenic mouse model with adipose tissue-specific endotrophin expression. We found that local endotrophin expression stimulates fibrosis by upregulating ECM constituents, both in an acute setting and also during a more chronic exposure. Through its chemoattractant action, it induces macrophage accumulation in adipose tissue [33] , leading to an overall more enhanced pro-inflammatory reaction in adipose tissue. Both the pro-fibrotic and pro-inflammatory effects contribute to the metabolic dysfunction of adipose tissue, which in turn triggers systemic insulin resistance. Of note, these findings demonstrate that adipocyte-derived endotrophin exerts local effects in adipose tissue independent of the tumour environment. Recently, a wide range of protein factors, which are collectively referred to as ‘adipokines’ have been identified in WAT, suggesting adipose tissue is an active secretary and endocrine organ, which is integrated into systemic physiological and metabolic control [2] , [3] , [34] , [35] . The adipokines encompass a wide range of metabolic functions, including the regulation of insulin sensitivity, food intake and energy balance, angiogenesis, inflammation and widespread involvement in the immune response [34] , [36] , [37] . Some adipokines, such as adiponectin and leptin, exert many of their functions through endocrine actions. On the other hand, other factors, such as TNFα, have a strong local impact based on their autocrine or paracrine actions [2] , [3] , [38] , [39] , [40] . Despite these apparent differences, a common aspect of these adipokines is that their levels are subject to stringent regulation under different metabolic conditions and their regulation is accompanied by changes in circulating inflammatory cytokines and acute-phase proteins [3] , [41] . As a novel adipocyte-derived factor, endotrophin can be efficiently cleaved and released from its parental COL6α3 chain. It can function either locally in adipose tissue to trigger fibrosis, inflammation and unfavourable metabolic effects as we found in this report; or more distally in tumour tissues to promote tumour progression [22] . Moreover, its levels are upregulated in both genetically challenged ob/ob mice and in obese subjects [22] . Our results demonstrate that local endotrophin overexpression potently induces a fibrotic microenvironment in adipose tissue by upregulating collagens, collagen cross-linking enzymes LOX and additional ECM constituents. Consistent with the studies in tumours, some of these fibrotic actions may be exerted through an upregulation of the TGF-β pathway. The functions of endotrophin could be via direct action on myofibroblast accumulation, differentiation or activation in fat tissue. TGF-β signalling components are upregulated in the transgenic mice. The TGF-β pathway is a well-established mediator of ECM deposition [42] . The pro-fibrotic actions of endotrophin could be inhibited with a neutralizing TGFβ antibody in the context of tumour invasion [22] . In addition, the increased levels of many collagens that are upregulated in the endotrophin transgenic fat pads could also contribute to an increased level of integrin signalling, which can in turn contribute to the metabolically unfavourable environment observed in fibrotic fat pads. Both acute and chronic collagen deposition during DIO development attract macrophage accumulation in adipose tissue [29] , [33] . Particularly, Henegar et al. [8] showed that fibrotic genes are upregulated in concert with pro-inflammatory genes upon analysis of the transcriptomic signature of WAT in obese individuals. Key studies by Cinti et al. [43] and by Obin et al. [33] indicate that macrophages aggregate surrounding the dead adipocytes in the obese fat pads to form CLS. The remnant lipid droplets left behind upon an adipocyte’s demise have to be cleared by macrophages. These macrophages are further activated and secrete pro-inflammatory factors that include IL-6, TNFα and MCP-1, and these inflammatory factors, when generated in excess, are implicated in the local processes that ultimately lead to the development of insulin resistance [1] , [41] , [44] , [45] , [46] . Many of these phenomena are recapitulated by endotrophin, even in the absence of a HFD challenge. This is apparent due to macrophages that infiltrate adipose tissue and cause inflammation as judged by the upregulation of F4/80 and SAA3 markers and the increased presence of CLS. As noted above, in both acute and chronic endotrophin induction models, we found the concomitant upregulation of pro-fibrotic and pro-inflammatory genes. Currently, we cannot determine whether there is a cause and effect relationship between the two or whether these processes occur in parallel in the context of a local elevation of endotrophin in fat tissue. Compared with a normal growing fat pad, an ‘unhealthy’ expansion includes a disproportionate enlargement of adipocytes, local hypoxic conditions and the induction of a fibrotic phenotype [1] . These conditions ultimately lead to an inflammatory phenotype that is tightly associated with systemic insulin resistance [47] , [48] . In ‘unhealthy’ fat pads, once a significant local level dysfunction limits the ability of adipose tissue to effectively take up and esterify free fatty acids, lipids start to ectopically build up in other tissues/organs via circulation. These ectopic fat deposits further promote insulin resistance [26] , [49] . Indeed, adipose tissue with elevated endotrophin levels leads rapidly to dysregulation of circulating triglycerides and free fatty acids, and eventually to hepatic steatosis. Through a mechanism that is not yet worked out, the endotrophin-mediated changes in adipose tissue trigger reduced energy expenditure without an effect on food intake, hence triggering an increase in fat mass and overall weight. This could also relate to the observation that endotrophin-induced fibrosis leads to local dysfunction in BAT as well, which as a result may be a mediator for the impaired ability for energy expenditure. From a therapeutic perspective, we consider the results presented on the effects of the endotrophin-neutralizing antibody to be most relevant. To test the specific pro-fibrotic and pro-inflammatory effects of endotrophin that lead to insulin resistance in obese fat pads, we injected a monoclonal anti-endotrophin antibody into HFD-challenged mice. Of note is the fact that we do this in wild-type mice, targeting endogenous endotrophin, not transgenically overproduced endotrophin. Surprisingly, the antibody treatment is effective not only while the mice are starting to experience the effects of the HFD but also significant improvements can be seen even upon initiating the treatment on the chronically challenged HFD mice. We have previously demonstrated that this antibody efficiently neutralizes endotrophin activity [22] . Although antibody injections did not prompt significant weight loss, it reduced fibrosis and led to a significant improvement in insulin sensitivity as judged by hyperinsulinemic–euglycemic clamp studies [22] . We have previously demonstrated that this neutralizing monoclonal anti-endotrophin antibody suppresses tumour growth in MMTV-PyMT mice [22] , and it also leads to substantial chemosensitization in the context of mammary tumours [23] . This further supports our notion that endotrophin is an important therapeutic target, both in the context of tumour studies as well as in the context of obesity-associated insulin resistance [22] . Even though we demonstrate the local pro-fibrotic and pro-inflammatory properties of endotrophin in adipose tissue along with a fair amount of insight into the functional consequences of excess local ‘hyperendotrophinemia’, two physiologically important questions still remain unresolved: First, what is the nature of the receptor(s) on the cell surface that mediate endotrophin action, and what are the downstream pathways that are endotrophin responsive, leading to the established pro-fibrotic and pro-inflammatory reactions in the adipocytes? Second, which specific MMPs are involved in the maturation of the endotrophin molecule, including its cleavage from its parental COL6α3 chain and where exactly is the endogenous cleavage site? Answers to both of the questions will help us to better understand the mechanisms by which endotrophin exerts its functions in both adipose tissue and tumours, ultimately creating a highly unfavourable microenvironment for metabolic flexibility. However, we appreciate that this upregulation of endotrophin can be seen in human adipose tissue as well, and within the tissues examined, endotrophin accumulates in distinct locations most likely outside the plasma membrane in the ECM, with little or no overlap with other markers examined, including the rest of the parental COL6 molecule. Animals To generate a Dox-inducible endotrophin overexpression mouse model (TRE-endotrophin), the complementary DNA encoding the murine COL6A3-C5 domain (amino acids 2590–2657, NP_034056) was fused to a stretch encoding the prolactin signal sequence at the N terminus, which allows endotrophin to be secreted from the cells [22] . This construct was cloned into the pTRE vector (Clontech). To better stabilize the transcript and enhance the translation, a Kozak sequence 5′-GCCGCCACC-3′ was inserted in front of the start codon and the rabbit β-globin 3′UTR was introduced into the 3′ end of the vector [25] . After linearization, TRE-endotrophin DNA was injected to embryos of a C57BL/6 background by the Transgenic Core Facility at UT Southwestern Medical Center. Adiponectin promoter-driven-rtTA transgenic mice (Apn-rtTA) were on a pure C57BL/6 background and have previously been described [24] . The characterization of the adiponectin promoter as a transgenic cassette has been described elsewhere [24] . These mice were crossed with TRE-endotrophin mice to generate the adipose tissue-specific Dox-inducible endotrophin transgenic mice. All experiments were conducted using littermate-controlled male mice and were started when these mice were 7 weeks old. Mice were housed in cages with 12-h dark–light cycle with free access to water and regular chow diet (cat. no. 5080; Labdiet, Frenchtown, NJ). All animal study protocols were approved by the Institutional Animal Care and Use Committee at University of Texas Southwestern Medical Center. HFD and dox containing HFD For all the HFD-feeding experiments, mice were fed with a diet containing 60% calories from fat (cat. no. D12492; Research Diets or Harlan, Madison, WI). The HFD paste with 600 mg kg −1 Dox also contains 60% calories from fat (cat. no. S5867; Bio-Serv, Frenchtown, NJ). Antibody neutralization The neutralizing monoclonal antibodies targeting mouse endotrophin, clone 10B6 (ref. 22 ) or IgG control (100 μg per mouse) were administrated by i.p. injection twice weekly for 4 weeks. Indirect calorimetric measurements For the metabolic cage studies, mice were housed individually in metabolic chambers and maintained on a 12-h dark–light cycle with lights on from 7:00 to 19:00 at room temperature (20~22 °C). Metabolic profiles were obtained continuously using TSA metabolic chambers (TSA System, Germany) in an open circuit indirect calorimetric system. All endotrophin transgenic mice and their littermate controls were also provided with HFD paste containing 200 mg kg −1 Dox and water ad libitum. Histology Adipose and liver tissues were excised and fixed in PBS buffered 10% formalin for 2 days. Following paraffin embedding, the tissue sections were stained with hematoxylin and eosin (H&E) and Masson's trichrome using standard protocols. For immunohistochemistry, sections were deparaffinized. After antigen retrieval and blockage of endogenous peroxidase, sections were stained with primary antibodies against endotrophin [22] (1:1,000, non-purified), F4/80 (0.1 mg ml −1 , 1:100; Santa Cruz, CA) and Mac-2 (1 mg ml −1 , 1:1,000; Tebu-Bio, France) followed by biotinylated secondary antibodies (0.85 mg ml −1 , 1:1,000 anti-rat; 0.5 mg ml −1 , 1:1,000 anti-mouse and 1.1 mg ml −1 , 1:1,000 anti-rabbit, respectively) (Dako, Glostrup, Denmark). Secondary antibodies were detected using DAB chromogen A kit (Dako) following the company’s protocol. The slides were also counterstained with hematoxylin. All the images were acquired with the Coolscope microscope (Nikon, Japan). Quantification of adipocyte diameters was done on H&E stained sections by the ImageJ software from the NIH ( http://rsbweb.nih.gov/ij/download.html ). Quantification of the blue colour density for the Masson’s trichrome staining was also done by ImageJ software. Liver lipid assays Frozen liver tissues were used for lipid extraction and measurement by the UT Southwestern Medical Center Metabolic Core Facility. In brief, ~100–150 mg frozen liver chunks were homogenized. Lipids were then extracted by the Folch procedure [50] and the chloroform phase was adjusted to equal volume, and triplicates of the samples in combination with standards, were dried down by the addition of 10 ml of 2:1 chloroform–Triton X-100 mix. Triglyceride and cholesterol levels were then assayed using Infinity reagent (Thermo Fisher Scientific, Waltham, MA). Systemic metabolic tests and blood chemistry For the OGTTs, mice were fasted for 3 h before administration of glucose (2.5 g kg −1 body weight; cat. no. 152527; MP Biomedicals) by gastric gavage. At the indicated time points, venous tail blood samples were collected by heparin-coated capillary tubes. Glucose levels were measured by an oxidase-peroxidase method with an assay kit (Sigma-Aldrich). For the ITTs, mice were fasted for 3 h before i.p. injection of insulin (0.75 unit per kg body weight; Novo Nordisk). At the indicated time points, venous tail blood samples were drawn by heparin-coated capillary tubes for glucose level measurements. Serum TG and FFA levels were measured by the kits following the protocols from the companies (Infinity; Thermo Fisher Scientific, Waltham, MA) (NEFA-HR(2); Wako Pure Chemical Industries, Tokyo, Japan). Protein analysis Total proteins were extracted from different adipose tissues with the methods described previously [29] . The protein concentration was measured with a BCA assay kit (Thermo Fisher Scientific, Rockford, IL). Proteins were then separated by denaturing and reducing SDS–polyacrylamide gel electrophoresis on 10% or 4–12% Bis-Tris gels (Invitrogen) and transferred to a PVDF membrane (Millipore Corp, Temecula, CA). For immunoblotting, the primary antibodies for adiponectin [51] were used followed by secondary antibodies labelled with infrared dye emitting at 800 nm (Li-Cor Bioscience). The blots were analysed with Odyssey software (version 2.1, Li-Cor Bioscience). Serum adiponectin levels were analysed by immunoblotting with the method above. In addition, serum leptin levels were measured by ELISA with a kit from Millipore. Quantitative real-time PCR Tissues excised from experimental mice were quickly frozen in liquid nitrogen. Total RNAs were extracted in Trizol (Invitrogen, Carlsbad, CA) using a TissueLyser (Qiagen, Valenica, CA) and then isolated with the RNeasy RNA extraction kit (Qiagen) following the company’s protocol. The purity and quantity of the mRNAs were determined by absorbance at 260/280 nm. cDNAs were prepared by reverse transcribing 500 ng of total mRNAs with a kit containing Superscript III reverse transcriptase and oligo (dT) 20 (Bio-Rad). qPCR reactions were carried out on an ABI Prism 7900 HT sequence detection system (Applied Biosystems). The relative amount of all mRNAs was calculated by using the comparative threshold cycle ( C T ) method. The housekeeping genes HPRT or GAPDH were used as the invariant control. Primer sequences are listed in Supplementary Table 1 . Confocal immunofluorescence imaging of human adipocytes A subcutaneous abdominal adipose tissue biopsy was obtained from the lateral part of the periumbilical area [52] from a healthy, overweight Caucasian male after an overnight fast. Small pieces of adipose tissue were fixed in 2% formaldehyde plus 0.15% picric acid at room temperature for 45 min, placed at 4 °C overnight for continued fixation, transferred to 50% glycerol and stored at −20 °C. The individual provided written informed consent before taking part in the study. The study adhered to the Helsinki II declaration, was approved by The Committees of Biomedical Research Ethics for the Capital Region in Denmark (H-4-2009-089) and registered at the Danish Data Protection Agency (2009-41-3682). For immunocytochemical analysis, small clusters of glycerol stored adipocytes were stained overnight with primary antibodies as described previously for muscle fibres [53] followed by Alexa 488- and Alexa 568-labelled secondary antibodies (Invitrogen, used at 3 μg ml −1 ), whole mounted in Vectashield (Vector Laboratories) and imaged on a confocal LSM 780 microscope (Zeiss). As primary antibodies, the following preparations were used: monoclonal antibody 5C6 directed against pan-COL6 (used at 1 μg ml −1 ) was obtained from the Developmental Studies Hybridoma Bank (University of Iowa), the anti-adiponectin (sc-136131, used at 1 μg ml −1 ) and anti-caveolin 1 (sc-53564, used at 1 μg ml −1 ) antibodies were from Santa Cruz, anti-leptin (#10221-MM01, used at 2 μg ml −1 ) was from Sino Biological, anti-BiP (SPA-827, used at 2 μg ml −1 ) was from Stressgen, anti-GLUT4 (F-27, used at 0.4 μg ml −1 ) was from Novo Nordisk and anti-IRAP (#6918, used at 1:250) was from Cell Signaling. A rabbit polyclonal anti-human endotrophin antibody was raised as a GST-fusion protein and used at 1:500 of crude serum. Human adipose tissue collection Omental adipose tissue specimens were obtained from 31 patients (female=22) undergoing laparoscopic Roux-en-Y gastric bypass. Seven of these patients (female=5) had type 2 diabetes mellitus, requiring treatment with metformin, insulin, thiazolidinedione, sulfonylurea, exenatide and/or dipeptidyl peptidase-4 inhibitor. The mean age of the cohort was 47 years (range 25–63 years) and the mean body mass index was 45 kg m −2 (range 35–71). Insulin responsiveness of total 31 obese patients is determined by HOMA2-IR values, which are divided in 3 groups; group 1 (<1.7), group 2 (1.7<and >2.6) and group 3 (>2.6). Group 1 is considered insulin sensitive (IS, n =9) and group3 is insulin resistance (IR, n =11). Groups 1 and 3 are comparable for BMI, age and glycaemia. There is no difference between the two groups in the number of diabetics. Quantification for ETP staining for each group is represented as mean ± s.d. Total 3–4 different fields of images per individuals were taken and quantified for staining positive area. After an overnight fast, the preoperative serum levels of insulin and glucose were determined. The homoeostatic model assessment of insulin resistant, updated version (HOMA2-IR), was used to estimate insulin resistance (available from www.dtu.ox.ac.uk ) using fasting glucose and fasting insulin levels. Samples of omental adipose tissue were immediately fixed in 10% buffered formalin after removal and embedded in paraffin from which multiple 5-μm sections were obtained. All subjects provided written informed consent before taking part in the study. The University of Massachusetts Medical School Institutional Review Board approved the study. Statistical analysis All the results are presented as means±s.e.m. or±s.d. Differences between two groups were determined for statistical significance by a standard two-tailed Student’s t-test . Differences between multiple groups were also determined by a two-way analysis of variance. Significance was accepted at a P- value of <0.05. How to cite this article: Sun, K. et al. Endotrophin triggers adipose tissue fibrosis and metabolic dysfunction. Nat. Commun. 5:3485 doi: 10.1038/ncomms4485 (2014).